BRMS1L suppresses breast cancer metastasis by inducing epigenetic silence of FZD10 BRMS1L (breast cancer metastasis suppressor 1 like, BRMS1-like) is a component of Sin3A–histone deacetylase (HDAC) co-repressor complex that suppresses target gene transcription. Here we show that reduced BRMS1L in breast cancer tissues is associated with metastasis and poor patient survival. Functionally, BRMS1L inhibits breast cancer cells migration and invasion by inhibiting epithelial–mesenchymal transition. These effects are mediated by epigenetic silencing of FZD10, a receptor for Wnt signalling, through HDAC1 recruitment and histone H3K9 deacetylation at the promoter. Consequently, BRMS1L-induced FZD10 silencing inhibits aberrant activation of WNT3-FZD10-β-catenin signalling. Furthermore, BRMS1L is a target of miR-106b and miR-106b upregulation leads to BRMS1L reduction in breast cancer cells. RNA interference-mediated silencing of BRMS1L expression promotes metastasis of breast cancer xenografts in immunocompromised mice, whereas ectopic BRMS1L expression inhibits metastasis. Therefore, BRMS1L provides an epigenetic regulation of Wnt signalling in breast cancer cells and acts as a breast cancer metastasis suppressor. Approximately 15% of breast cancer patients develop disseminated metastasis before or after diagnosis, and distant metastasis is responsible for around 90% of breast cancer-associated mortality [1] . Therefore, it is necessary to understand the mechanisms that underlie breast cancer metastasis. A large number of metastasis-associated genes have been shown to participate in regulating multiple processes of cancer metastasis. Repression of metastasis-associated genes at transcription level has a significant role in suppressing breast cancer progression and metastasis, which is partly mediated by recruitment of repressor or co-repressor complexes that contain histone deacetylase (HDAC) to their promoters [2] , [3] , [4] . Among these complexes, the core switch-independent 3 (SIN3)–HDAC complex that integrates a wide variety of repressors and co-repressors are important inhibitors for cancer progression [5] , [6] . SIN3 is a scaffolding protein that was initially identified as a global regulator of gene transcription in yeast, whereas two isoforms have been found in mammals, Sin3A and Sin3B [7] , [8] . SIN3 proteins can link HDAC and co-repressors to chromatin-bound transcription factors to inhibit target gene expression [9] , [10] . Downregulation of breast cancer metastasis suppressor 1 (BRMS1), a major co-repressor interacting with Sin3A, is associated with metastasis of multiple types of malignancies, including breast, nasopharyngeal, melanoma, non-small-cell lung cancinomas and melanomas [11] , [12] , [13] , [14] , [15] . Moreover, transfection of BRMS1 into highly metastatic human breast cancer cell lines significantly inhibited lung metastasis in xenografted mice without influencing orthotopic tumour incidence and growth rate, suggesting that BRMS1 is a metastasis suppressor [16] . It has been shown that BRMS1 inhibits invasion, migration and adhesion of breast cancer cells and promote their apoptosis, suggesting that it acts on multiple steps in the metastatic cascade [15] , [16] , [17] , [18] . Further, mechanistic studies have revealed that in association with SIN3 and HDAC1/2, BRMS1 transcriptionally represses a panel of metastasis-associated target genes, including osteopontin [19] , [20] , urokinase-type plasminogene activator [21] , EGFR [22] , CXCR4 (ref. 23 ) and a number of metastasis-associated microRNAs (miRNAs) [24] , [25] , [26] , probably by modifying the overall composition of SIN3 complexes leading to changes in the specificity and activity of HDAC. In addition to BRMS1, several other co-repressors have been characterized as components of SIN3 complex. Among them, suppressor of defective silencing 3 and BRMS1-like (BRMS1L) share 23% and 57% identical amino-acid sequence, respectively, to BRMS1 as well as a conserved region of Sds3-like domain that is important for protein–protein interaction [27] . As BRMS1 gene is often deleted or epigenetically silenced in breast cancer, it is possible that structurally analogous proteins may provide functional compensation for BRMS1 in cancer suppression. However, overexpression of suppressor of defective silencing 3 does not suppress metastasis of human cancer cells, and it remains obscure whether BRMS1L may impact on breast cancer metastasis [28] . BRMS1L is a component recently purified from the Sin3A complex, which shares homology with the yeast and mammalian Sds3 proteins as BRMS1. Sin3A complex containing BRMS1L is capable of histone deacetylation and transcription suppression. Although the contribution of BRMS1L in cancer development is not well characterized, it was shown that BRMS1L inhibited the growth of a human lung cancer cell line [27] . In the present study, we demonstrated that BRMS1L suppresses breast cancer invasiveness and metastasis by inhibiting epithelial–mesenchymal transition (EMT) of the tumour cells. This effect is mediated by epigenetic silence of FZD10 gene via facilitating the recruitment of HDAC1 to its promoter to enhance histone H3K9 deacetylation. In addition, BRMS1L expression in primary tumours of breast cancer patients is associated with less lymph node and distant metastasis, as well as better clinical outcome. Reduced BRMS1L is associated with breast cancer metastasis Owing to high homology of BRMS1L with BRMS1, which suppresses breast cancer metastasis, we investigated whether the mRNA and protein expression of BRMS1L in 428 cases of primary breast cancer is associated with metastasis. Immunohistochemical staining for BRMS1L protein was much weaker and less extensive in nuclei and cytoplasm in the primary tumour cells of invasive breast cancer than normal breast tissues. In addition, BRMS1L protein level was much lower in primary breast cancer tissues with regional lymph node metastasis than those without. Furthermore, there were less signals observed in lymph node metastases and brain metastases compared with primary breast cancer tissues ( Fig. 1a ). Similarly, BRMS1L mRNA level, determined by quantitative reverse transcription–PCR (qRT–PCR), was much lower in primary breast cancer tissues with regional lymph node metastases and liver metastasis than those without metastasis ( P ≪ 0.001, t -test, Fig. 1b ). 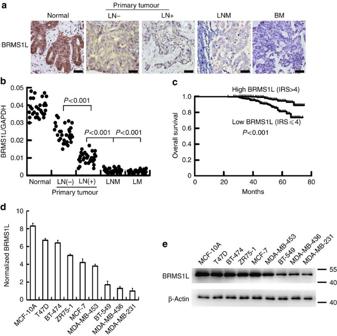Figure 1: BRMS1L expression in breast tissues and cell lines. (a) Representative immunohistochemical staining of BRMS1L in normal breast tissue (normal), primary breast cancer with or without regional lymph node (LN) metastasis, metastatic lymph nodes (LNM) and brain metastases (BM). Scale bar corresponds to 50 μm. (b) The ratio of BRMS1L versus gyceraldehyde 3-phosphate dehydrogenase (GAPDH) mRNA measured by qRT–PCR in normal breast tissue (normal;n=30), primary breast cancer with (n=30) or without regional LN metastasis (n=30), LNM (n=30) and liver metastases (LM; =30). Student’st-test was used for the comparison of two independent groups. (c) Kaplan–Meier overall survival (OS) curve of patients with low (IRS≤4) and high (IRS>4) BRMS1L levels with a median follow-up period of 55 months. Log Rank Test was used to analyse survival differences. (d,e) mRNA and protein expression levels of BRMS1L measured by qRT–PCR (d) and western blotting (e) in various breast epithelial cell lines. Bars correspond to mean±s.d. These data are representative of three independent experiments. Figure 1: BRMS1L expression in breast tissues and cell lines. ( a ) Representative immunohistochemical staining of BRMS1L in normal breast tissue (normal), primary breast cancer with or without regional lymph node (LN) metastasis, metastatic lymph nodes (LNM) and brain metastases (BM). Scale bar corresponds to 50 μm. ( b ) The ratio of BRMS1L versus gyceraldehyde 3-phosphate dehydrogenase (GAPDH) mRNA measured by qRT–PCR in normal breast tissue (normal; n =30), primary breast cancer with ( n =30) or without regional LN metastasis ( n =30), LNM ( n =30) and liver metastases (LM; =30). Student’s t -test was used for the comparison of two independent groups. ( c ) Kaplan–Meier overall survival (OS) curve of patients with low (IRS≤4) and high (IRS>4) BRMS1L levels with a median follow-up period of 55 months. Log Rank Test was used to analyse survival differences. ( d , e ) mRNA and protein expression levels of BRMS1L measured by qRT–PCR ( d ) and western blotting ( e ) in various breast epithelial cell lines. Bars correspond to mean±s.d. These data are representative of three independent experiments. Full size image Next we analysed the association between BRMS1L expression and the clinicopathological status of 428 breast cancer patients ( Supplementary Table 1 ). The expression of BRMS1L was associated with smaller tumour size ( P =0.005, Supplementary Table 1 ), lower clinical stage ( P =0.021, χ 2 -test, Supplementary Table 1 ), less positive lymph node ( P ≪ 0.001, χ 2 -test, Supplementary Table 1 ) and less distant metastasis ( P ≪ 0.001, χ 2 -test, Supplementary Table 1 ). However, there was no correlation between BRMS1L expression and patient age, histological grade, estrogen receptor or Her2 status ( Supplementary Table 1 ). Moreover, the Kaplan–Meier survival curve with a median follow-up of 55 months demonstrated that patients with high BRMS1L expression (immunoreactive score, IRS>4) had a longer overall survival ( P ≪ 0.001, Log rank test , Fig. 1c ) than those with low BRMS1L expression (IRS≤4). 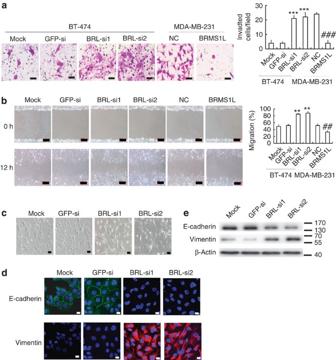Figure 2: BRMS1L suppresses breast cancer migration and invasion. (a) Invasion of cancer cells measured by Boyden chamber assays in BT-474 cells that were mock transfected (mock), or transfected with GFP-siRNA or either of the two BRMS1L-siRNAs (BRL-si1 and BRL-si2) and in MDA-MB-231 cells transfected with a pcDNA3 vector carrying BRMS1L (BRMS1L) or an empty vector as negative control (NC). Scale bars correspond to 50 μm. Bars correspond to mean±s.d. ***P≪0.001 as compared with GFP-siRNA.###P≪0.001, as compared with NC. Student’st-test was used for the comparison of two independent groups. (b) Wound-healing assay for MDA-MB-231 cells that were mock transfected (mock), or transfected with GFP-siRNA, BRMS1L-siRNAs, pcDNA3 vector carrying BRMS1L (BRMS1L) or negative control (NC). Bars correspond to mean±s.d. **P≪0.01 as compared with GFP-siRNA.##P≪0.01, as compared with NC. Scale bar corresponds to 200 μm. Student’st-test was used for the comparison of two independent groups. (c–e) Phase-contrast microscopy (c), immunofluorescent staining (d) and western blotting (e) for MCF-10A that were mock transfected, or transfected with GFP-siRNA or BRMS1L-siRNAs. Scale bars correspond to 50 μm. BRL, BRMS1L. In addition, multivariate Cox hazard analysis demonstrated that BRMS1L expression was an independent prognostic factor of overall survival ( Supplementary Table 2 ). 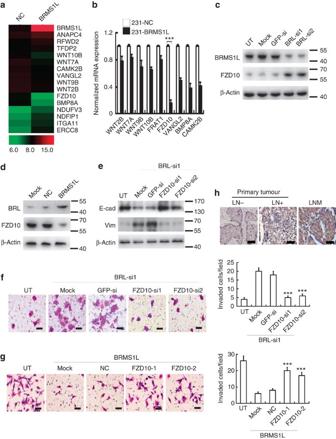Figure 3: BRMS1L inhibits breast cancer cell invasion and EMT via suppressing FZD10 expression. (a) mRNA microarray (GSE61354) analysis reveals mRNA differentially expressed in MDA-MB-231 cells transfected with pcDNA3 vector carrying BRMS1L (BRMS1L) or negative control (NC) for 24 h. (b) qRT–PCR for the mRNA expression ofWNT2B,WNT7A,WNT9B,WNT10B,FRAT1,FZD10,VANGL2,BMP8A,CAMK3Bin mRNA microarray. ***P≪0.001 as compared with NC. Bars correspond to mean±s.d. The data are representative of three independent experiments. Student’st-test was used for the comparison of two independent groups. (c) Western blotting for BRMS1L and FZD10 in T47D cells that were untreated (UT), mock transfected (mock) or transfected with GFP-siRNA or two BRMS1L-siRNAs. (d) Western blotting for BRMS1L and FZD10 in MDA-MB-231 cells that were transfected with pcDNA3 vector carrying BRMS1L (BRMS1L) or negative control (NC). (e) E-cadherin and vimentin protein expression levels measured by western blotting in MCF-10A cells that were untreated (UT), mock transfected (mock) or transfected with GFP-siRNA or two FZD10-siRNAs. (f,g) Invasion of cancer cells measured by Boyden chamber assays for BT-474 (f) and MDA-MB-231 cells (g) treated as indicated. Bars correspond to mean±s.d. ***P≪0.001 as compared with mock. Scale bars correspond to 50 μm. Student’st-test was used for the comparison of two independent groups. (h) Immunohistochemical staining for FZD10 in primary breast cancer with or without regional lymph nodes (LN) metastasis and metastatic lymph nodes (LNMs). Scale bar corresponds to 50 μm. BRL, BRMS1L; E-cad, E-cadherin; Vim, Vimentin. These findings were verified by Oncomine database with three independent data sets including a TCGA data set (593 cases) demonstrating that BRMS1L expression is lower in breast cancer than in normal breast tissues and decreased BRMS1L is associated with poor prognosis of breast cancer patients ( Supplementary Table 3 ). Collectively, these data suggest that BRMS1L reduction is related to clinical metastasis and poor prognosis of breast cancer. In addition, we examined BRMS1L mRNA and protein expression in several breast cancer cell lines with epithelial or mesenchymal phenotype. Interestingly, BRMS1L mRNA was much lower in mesenchymal-like breast cancer lines (MDA-MB-231 and MDA-MB-436) than in epithelial cancer lines (T47D, BT-474 and MCF-7) and nontumorigenic MCF-10A breast epithelial cell line ( Fig. 1d ). Likewise, the protein level of BRMS1L was much higher in epithelial breast cancer lines than in mesanchymal-like ones ( Fig. 1e ). Therefore, our data suggest that like BRMS1, reduced BRMS1L expression maybe associated with EMT of breast cancer cells, which is related to their metastatic potential. BRMS1L inhibits invasion by inhibiting EMT To evaluate whether BRMS1L regulates the invasiveness of breast cancer cells, we employed Boyden chamber assays by plating cancer cells on inserts coated with Matrigel. Transfection efficiency of the two BRMS1L-siRNAs and the pcDNA3 vector carrying BRMS1L was measured by western blotting ( Supplementary Fig. 1a and b ). Silencing BRMS1L expression in BT-474 cells with high endogenous BRMS1L level using two different BRMS1L-siRNAs increased the number of invaded cancer cells by 5.25- and 5.5-fold, respectively ( P ≪ 0.001, Fig. 2a ). In contrast, ectopic expression of BRMS1L in MDA-MB-231 cells with low BRMS1L level reduced the invaded cells by 83% ( P ≪ 0.001, Fig. 2a ). Similarly, Boyden chamber assay without Matrigel coating or wound-healing assay showed that silencing or enforcing BRMS1L expression in breast cancer cells enhanced or inhibited their migration, respectively ( Supplementary Fig. 1c and 2b ). Collectively, these data suggest that BRMS1L suppresses the invasiveness and motility of breast cancer cells. Figure 2: BRMS1L suppresses breast cancer migration and invasion. ( a ) Invasion of cancer cells measured by Boyden chamber assays in BT-474 cells that were mock transfected (mock), or transfected with GFP-siRNA or either of the two BRMS1L-siRNAs (BRL-si1 and BRL-si2) and in MDA-MB-231 cells transfected with a pcDNA3 vector carrying BRMS1L (BRMS1L) or an empty vector as negative control (NC). Scale bars correspond to 50 μm. Bars correspond to mean±s.d. *** P ≪ 0.001 as compared with GFP-siRNA. ### P ≪ 0.001, as compared with NC. Student’s t -test was used for the comparison of two independent groups. ( b ) Wound-healing assay for MDA-MB-231 cells that were mock transfected (mock), or transfected with GFP-siRNA, BRMS1L-siRNAs, pcDNA3 vector carrying BRMS1L (BRMS1L) or negative control (NC). Bars correspond to mean±s.d. ** P ≪ 0.01 as compared with GFP-siRNA. ## P ≪ 0.01, as compared with NC. Scale bar corresponds to 200 μm. Student’s t -test was used for the comparison of two independent groups. ( c – e ) Phase-contrast microscopy ( c ), immunofluorescent staining ( d ) and western blotting ( e ) for MCF-10A that were mock transfected, or transfected with GFP-siRNA or BRMS1L-siRNAs. Scale bars correspond to 50 μm. BRL, BRMS1L. Full size image Further, we investigated whether BRMS1L expression influences the EMT of breast epithelial cells. Knockdown of BRMS1L by siRNAs in MCF-10A, a nontumorigenic breast epithelial cell line, resulted in prominent morphological changes of the cells from a rounded or polygonal, epithelial-like form to an elongated or spindle-shaped, mesenchymal form ( Fig. 2c ). The morphological changes of MCF-10A cells with BRMS1L silencing were accompanied by reduced E-cadherin and marked induction of Vimentin ( Fig. 2d and e ). In contrast, ectopic expression of BRMS1L tended to change the morphology of MDA-MB-231 cells from the spindle and elongated mesenchymal form to more rounded and polygonal epithelial-like form. Moreover, BRMS1L reduced the mRNA level of fibronectin and vimentin ( Supplementary Fig. 1d and 1e ), two major markers of mesenchymal phenotype. Therefore, reduced BRMS1L expression enhances the invasiveness of breast cancer cells probably by inducing EMT, whereas overexpressing BRMS1L may reverse EMT in the tumour cells. BRMS1L inhibits EMT by suppressing FZD10 expression As BRMS1L is a component of the Sin3A co-repressor complex, we employed mRNA microarray to explore the target genes that BRMS1L modulated to inhibit EMT and invasiveness of breast cancer cells. To identify target genes that are regulated by BRMS1L, mRNA microarray was done for MDA-MB-231 cells before and after transient transfection of a BRMS1L-expressing pcDNA3 vector or an empty vector as negative control. After hierarchical clustering ( Fig. 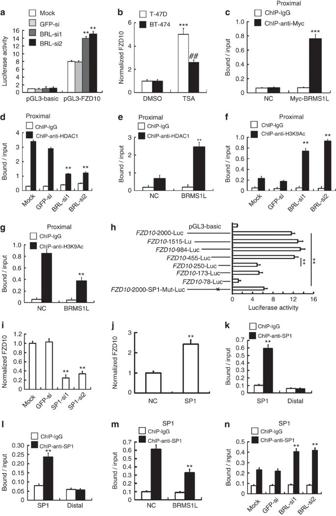Figure 4: BRMS1L reduces acetylated H3K9 level ofFZD10promoter and suppresses SP1-mediatedFZD10transcription. (a) T47D cells with stable transfection of pGL3-FZD10 promoter were transfected with BRMS1L-siRNAs or GFP-siRNA and assayed for luciferase activity. **P≪0.01 as compared with GFP-siRNA. (b) qRT–PCR forFZD10mRNA expression normalized to GAPDH in T47D and BT-474 cells treated with 200 ng ml−1trichostatin A (TSA) for 24 h. **P≪0.01,##P≪0.01 as compared with dimethylsulphoxide (DMSO). (c) ChIP analysis for BRMS1L binding toFZD10promoter in MDA-MB-231 cells transfected with Myc-BRMS1L or negative control (NC). Enrichment of promoter region was normalized by input. ***P≪0.001 as compared with NC. (d,e) ChIP analysis for HDAC1 binding toFZD10promoter in T47D cells transfected with BRMS1L-siRNAs or GFP-siRNA (d) and in MDA-MB-231 cells transfected with pcDNA3 vector carrying BRMS1L (BRMS1L) or negative control (NC) (e). Enrichment of promoter region was normalized by input. **P≪0.01 as compared with GFP-siRNA or NC. (f,g) ChIP analysis for H3K9Ac binding toFZD10promoter in T47D cells transfected with BRMS1L-siRNAs or GFP-siRNA (f) and in MDA-MB-231 cells transfected with pcDNA3 vector carrying BRMS1L (BRMS1L) or negative control (NC; (g). Enrichment of promoter region was normalized by input. **P≪0.01 as compared with GFP-siRNA or NC. (h) Luciferase reporter assays for the truncated or mutantFZD10promoter constructs transfected in MDA-MB-231 cells. **P≪0.01. (i)FZD10mRNA normalized to GAPDH in MDA-MB-231 cells that were mock transfected (mock), or transfected with GFP-siRNA or two SP1-siRNAs. **P≪0.01 as compared with GFP-siRNA. (j)FZD10mRNA normalized to GAPDH in T47D cells that were transfected with pcDNA3 vector carrying SP1 (SP1) or negative control (NC). **P≪0.01 as compared with NC. (k,l) ChIP analysis for SP1 binding toFZD10promoter in MDA-MB-231 cells (k) and T47D cells (l). Enrichment of promoter region was normalized by input. **P≪0.01 as compared with anti-IgG. (m,n) ChIP analysis for SP1 binding to theFZD10promoter in MDA-MB-231 cells transfected with pcDNA3 vector carrying BRMS1L (BRMS1L) or negative control (NC;m) and in T47D cells transfected with BRMS1L-siRNAs or GFP-siRNA (n). Enrichment of promoter region was normalized by input. **P≪0.01 as compared with NC or GFP-siRNA. BRL, BRMS1L. Bars correspond to mean±s.d. These data are representative of three independent experiments. Student’st-test was used for the comparison of two independent groups. 3a ), the top 50 upregulated and downregulated genes were correlated to different signalling pathways ( Supplementary Table 4 ). Notably, BRMS1L significantly repressed the expression of a panel of genes in the Wnt signalling pathway, which have been associated with tumorigenesis [29] , EMT [30] and enhanced cancer invasiveness and metastasis [30] , [31] , [32] . Furthermore, qRT–PCR verified that WNT9B and WNT10B , two important Wnt ligands, were reduced by BRMS1L for 1.43- and 1.61-fold, respectively, whereas FZD10 (frrizled class receptor 10) , a Wnt signalling receptor [33] , [34] , [35] , was reduced by 84% ( P ≪ 0.001, t -test, Fig. 3b ). In addition, among all the FZD receptors for wnt signalling pathway, FZD10 was the only one with significant change following BRMS1L transfection ( Supplementary Fig. 2a and b , Supplementary Table 7 ). Figure 3: BRMS1L inhibits breast cancer cell invasion and EMT via suppressing FZD10 expression. 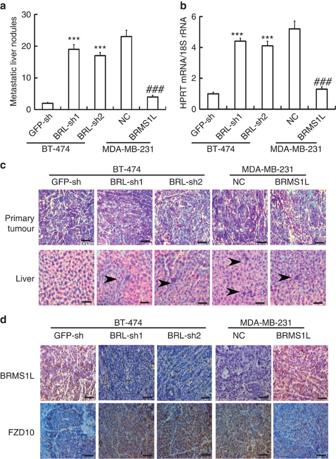Figure 7: BRMS1L inhibits liver metastasis of breast tumour xenografts without influencing orthotopic tumour incidence and growth rate. (a) The number of metastatic liver nodules in mice xenografted with breast cancer cells as indicated. The bars correspond to the mean±s.d. ***P≪0.001 compared with GFP-shRNA.###P≪0.001 as compared with NC (n=8 per group). Student’st-test was used for the comparison of two independent groups. (b) Expression of human HPRT mRNA relative to mouse 18S rRNA in the liver. Bars correspond to mean±s.d. Eight independent experiments were repeated (each mouse sample was considered as one independent experiment. Five technological replications were repeated in each sample.). Student’st-test was used for the comparison of two independent groups. (c) Haematoxylin and eosin (H&E) staining for tumour xenografts and liver metastases of mice xenografted with breast cancer cells as indicated. Scale bars correspond to 50 μm. (d) Immunohistochemical staining for BRMS1L and FZD10 expression in tumour xenografts of mice xenografted with breast cancer cells as indicated. Scale bars correspond to 50 μm.BRL, BRMS1L. ( a ) mRNA microarray (GSE61354) analysis reveals mRNA differentially expressed in MDA-MB-231 cells transfected with pcDNA3 vector carrying BRMS1L (BRMS1L) or negative control (NC) for 24 h. ( b ) qRT–PCR for the mRNA expression of WNT2B , WNT7A , WNT9B , WNT10B , FRAT1 , FZD10 , VANGL2 , BMP8A , CAMK3B in mRNA microarray. *** P ≪ 0.001 as compared with NC. Bars correspond to mean±s.d. The data are representative of three independent experiments. Student’s t -test was used for the comparison of two independent groups. ( c ) Western blotting for BRMS1L and FZD10 in T47D cells that were untreated (UT), mock transfected (mock) or transfected with GFP-siRNA or two BRMS1L-siRNAs. ( d ) Western blotting for BRMS1L and FZD10 in MDA-MB-231 cells that were transfected with pcDNA3 vector carrying BRMS1L (BRMS1L) or negative control (NC). ( e ) E-cadherin and vimentin protein expression levels measured by western blotting in MCF-10A cells that were untreated (UT), mock transfected (mock) or transfected with GFP-siRNA or two FZD10-siRNAs. ( f , g ) Invasion of cancer cells measured by Boyden chamber assays for BT-474 ( f ) and MDA-MB-231 cells ( g ) treated as indicated. Bars correspond to mean±s.d. *** P ≪ 0.001 as compared with mock. Scale bars correspond to 50 μm. Student’s t -test was used for the comparison of two independent groups. ( h ) Immunohistochemical staining for FZD10 in primary breast cancer with or without regional lymph nodes (LN) metastasis and metastatic lymph nodes (LNMs). Scale bar corresponds to 50 μm. BRL, BRMS1L; E-cad, E-cadherin; Vim, Vimentin. Full size image To confirm whether BRMS1L suppresses FZD10 expression, we silenced BRMS1L expression in epithelial-like T47D breast cancer cells or enforced BRMS1L expression in mesanchymal-like MDA-MB-231 cells. As expected, silencing of BRMS1L expression in T47D cells efficiently increased FZD10 mRNA and protein ( Fig. 3c and Supplementary Fig. 2c ). Further, ectopic expression of BRMS1L in MDA-MB-231 cells resulted in decreased FZD10 mRNA and protein expression ( Fig. 3d and Supplementary Fig. 2d ). Therefore, BRMS1L suppresses the mRNA and protein expression of FZD10. Next, we investigated whether BRMS1L-mediated FZD10 downregulation contributes to inhibition of EMT and invasiveness of breast epithelial cells. Although silencing BRMS1L led to EMT in MCF-10A cells with reduced E-cadherin and increased vimentin, co-transfection with FZD10-siRNA efficiently abolished the EMT induced by BRMS1L silencing ( Fig. 3e ). In addition, co-transfection with FZD10-siRNA efficiently alleviated the promoting effect of BRMS1L-siRNA on the invasion of MDA-MB-231 cells ( P ≪ 0.001, t -test, Fig. 3f ). Conversely, enforced expression of FZD10 gene abrogated BRMS1L-induced inhibition in invasion of MDA-MB-231 cells with ectopic BRMS1L expression ( P ≪ 0.001, t -test, Fig. 3g ). To further evaluate the clinical significance of BRMS1L-FZD10 signalling, we examined FZD10 expression in breast cancer tissues using immunohistochemistry (IHC) and correlated it with BRMS1L immunostaining. FZD10 expression was much higher in the primary tumours with axillary lymph nodes metastasis, and even higher in the metastatic lesions than the primary tumours ( Fig. 3h ). In addition, FZD10 expression in breast cancer was negatively associated with BRMS1L ( r =−0.762, P ≪ 0.001, linear regression, Supplementary Fig. 2e ). Furthermore, we found that FZD10 protein level was much higher in mesenchymal-like MDA-MB-231 and MDA-MB-436 cells than in epithelial T47D and BT-474 cells ( Supplementary Fig. 2f ), which is opposite to the BRMS1L pattern. To further confirm the BRMS1L–FZD10 relationship, we searched Oncomine database to analyse the correlations between BRMS1L and FZD10 expression in breast cancer. Four data sets showed that FZD10 expression is negatively correlated with BRMS1L ( Supplementary Table 3 ). In addition, oncomine database showed that triple negative breast cancers that tend to present stronger mesenchymal phenotype [36] and Wnt pathway activation [37] have higher FZD10 expression than other breast cancer subtypes ( Supplementary Table 3 ). Collectively, these data suggest that BRMS1L inhibits EMT and invasiveness of breast cancer cells via downregulation of FZD10. BRMS1L transcriptionally suppresses FZD10 via HDAC complex As BRMS1L has been shown to inhibit transcription of a luciferase reporter gene [27] , we investigated whether BRMS1L could suppress the transcriptional activity of FZD10 promoter. A DNA fragment between −2,000 to +50 relative to FZD10 transcription start site (TSS) was cloned into a pGL3-Basic plasmid to yield pGL3- FZD10 recombinant vector delivering FZD10 promoter. Consistent with the qRT–PCR and western blot results above, silencing BRMS1L significantly increased the luciferase activity of pGL3-FZD10 in T47D cells ( P ≪ 0.01, t -test, Fig. 4a ). However, ectopic expression of BRMS1L in MDA-MB-231 cells reduced luciferase activity of pGL3-FZD10 by 2.5-fold ( P ≪ 0.001, t -test, Supplementary Fig. 3a ). These data indicate that BRMS1L represses the transcriptional activity of FZD10 promoter. Figure 4: BRMS1L reduces acetylated H3K9 level of FZD10 promoter and suppresses SP1-mediated FZD10 transcription. ( a ) T47D cells with stable transfection of pGL3-FZD10 promoter were transfected with BRMS1L-siRNAs or GFP-siRNA and assayed for luciferase activity. ** P ≪ 0.01 as compared with GFP-siRNA. ( b ) qRT–PCR for FZD10 mRNA expression normalized to GAPDH in T47D and BT-474 cells treated with 200 ng ml −1 trichostatin A (TSA) for 24 h. ** P ≪ 0.01, ## P ≪ 0.01 as compared with dimethylsulphoxide (DMSO). ( c ) ChIP analysis for BRMS1L binding to FZD10 promoter in MDA-MB-231 cells transfected with Myc-BRMS1L or negative control (NC). Enrichment of promoter region was normalized by input. *** P ≪ 0.001 as compared with NC. ( d , e ) ChIP analysis for HDAC1 binding to FZD10 promoter in T47D cells transfected with BRMS1L-siRNAs or GFP-siRNA ( d ) and in MDA-MB-231 cells transfected with pcDNA3 vector carrying BRMS1L (BRMS1L) or negative control (NC) ( e ). Enrichment of promoter region was normalized by input. ** P ≪ 0.01 as compared with GFP-siRNA or NC. ( f , g ) ChIP analysis for H3K9Ac binding to FZD10 promoter in T47D cells transfected with BRMS1L-siRNAs or GFP-siRNA ( f ) and in MDA-MB-231 cells transfected with pcDNA3 vector carrying BRMS1L (BRMS1L) or negative control (NC; ( g ). Enrichment of promoter region was normalized by input. ** P ≪ 0.01 as compared with GFP-siRNA or NC. ( h ) Luciferase reporter assays for the truncated or mutant FZD10 promoter constructs transfected in MDA-MB-231 cells. ** P ≪ 0.01. ( i ) FZD10 mRNA normalized to GAPDH in MDA-MB-231 cells that were mock transfected (mock), or transfected with GFP-siRNA or two SP1-siRNAs. ** P ≪ 0.01 as compared with GFP-siRNA. ( j ) FZD10 mRNA normalized to GAPDH in T47D cells that were transfected with pcDNA3 vector carrying SP1 (SP1) or negative control (NC). ** P ≪ 0.01 as compared with NC. ( k , l ) ChIP analysis for SP1 binding to FZD10 promoter in MDA-MB-231 cells ( k ) and T47D cells ( l ). Enrichment of promoter region was normalized by input. ** P ≪ 0.01 as compared with anti-IgG. ( m , n ) ChIP analysis for SP1 binding to the FZD10 promoter in MDA-MB-231 cells transfected with pcDNA3 vector carrying BRMS1L (BRMS1L) or negative control (NC; m ) and in T47D cells transfected with BRMS1L-siRNAs or GFP-siRNA ( n ). Enrichment of promoter region was normalized by input. ** P ≪ 0.01 as compared with NC or GFP-siRNA. BRL, BRMS1L. Bars correspond to mean±s.d. These data are representative of three independent experiments. Student’s t -test was used for the comparison of two independent groups. Full size image Given that BRMS1L is known to repress transcriptional activity of gene promoters by associating with Sin3A-HDAC1/2 complex that mediates histone deacetylation [27] , we examined whether HDAC inhibition could affect FZD10 transcription in breast cancer cells with high BRMS1L expression. Treatment of T47D and BT474 cells with trichostatin A, a HDACs inhibitor significantly increased FZD10 mRNA expression by 5- ( P ≪ 0.001, t -test) and 2.5-fold ( P ≪ 0.01, t -test), respectively ( Fig. 4b ), suggesting that FZD10 transcription is regulated by histone deacetylation. We next investigated whether BRMS1L facilitates the recruitment of HDAC1/2 complex to FZD10 promoter and is responsible for its histone deacetylation. Chromatin immunoprecipitation (ChIP) assay was performed to evaluate binding of the BRMS1L and Sin3A–HDAC1/2 complex to FZD10 promoter. To confirm binding of BRMS1L complex to the FZD10 promoter, we expressed Myc-tagged BRMS1L into MDA-MB-231 cells and performed ChIP to examine the association of BRMS1L complex with FZD10 promoter. Anti-Myc antibody, but not the isotype IgG, efficiently retrieved the proximal region of FZD10 promoter in MDA-MB-231 cells ectopically expressing Myc-BRMS1L ( P ≪ 0.001, t -test, Fig. 4c ). However, anti-Myc antibody did not retrieve the distal region of FZD10 promoter ( Supplementary Fig. 3b and c ). Furthermore, we examined whether the existence of BRMS1L affects binding of HDAC1/2 complex to FZD10 promoter. Upon silencing BRMS1L in T47D cells, enrichment of FZD10 promoter proximal region by anti-HDAC1 antibody was dramatically reduced ( P ≪ 0.01, t -test, Fig. 4d ), whereas enforcing BRMS1L expression in MDA-MB-231 cells increased the enrichment of FZD10 promoter proximal region ( P ≪ 0.01, t -test, Fig. 4e ). To further investigate whether BRMS1L affects the deacetylation activity of HDAC1/2 complex, we performed ChIP assay with antibody against H3K9Ac, a substrate of HDAC1/2 deacetylase. Silencing BRMS1L in T47D cells increased anti-H3K9Ac-mediated enrichment of FZD10 promoter proximal region ( P ≪ 0.01, Fig. 4f ), whereas ectopic expression of BRMS1L in MDA-MB-231 cells reduced the enrichment ( P ≪ 0.01, t -test, Fig. 4g ). However, changing BRMS1L expression did not affect anti-HDAC1- or anti-H3K9Ac-mediated enrichment of FZD10 promoter distal region ( Supplementary Fig. 3d–g ), confirming the specificity of the above enrichment for FZD10 promoter proximal region. Therefore, these findings suggest that BRMS1L represses FZD10 transcription by facilitating the recruitment of the Sin3A–HDAC1/2 deacetylase suppressor complex to FZD10 promoter and thus reducing acetylation of HDAC1/2 substrates. BRMS1L antagonizes SP1-promoted FZD10 transcription We further explored the mechanism for enhanced FZD10 transcription in breast cancer cells with reduced BRMS1L expression and the contribution of BRMS1L in this scenario by transfecting MDA-MB-231 cells with pGL3 reporter plasmids that contain sequential deletions of the 5′-flanking region of FZD10 promoter. Sequence deletions from −2,000 bp up to −455 bp upstream of the TSS of FZD10 did not obviously influence the luciferase activities, but deletion to −250 bp significantly inhibited the activity ( Fig. 4h ), implying the presence of crucial regulatory elements between −455 and −250 bp in the promoter region of FZD10 . Deletion to −173 bp remained the luciferase activity similar as deletion to −250 bp, but deletion to −78 bp reduced the luciferase activity to similar level as pGL3-Basic control vector, indicating that −173/−78 region is responsible for the basal transcription of FZD10 in breast cancer cells ( Fig. 4h ). Sequence analysis with the MCatch software revealed a SP1-binding site located at −294 to −280 bp upstream of FZD10 TSS ( Supplementary Fig. 4a ), wherein its point mutations significantly reduced the luciferase activity to similar level as the deleted plasmid with only 250 bp upstream of FZD10 TSS ( Fig. 4h ). Therefore, an SP1-binding site was involved in the full transactivation activity in the FZD10 promoter region. To confirm whether SP1 regulates FZD10 transcription, we examined changes of FZD10 mRNA expression by silencing or overexpressing SP1 in breast cancer cells ( Supplementary Fig. 4b and c ). Indeed, silencing SP1 in MB-MDA-231 cells reduced FZD10 mRNA expression by approximately 70% ( Fig. 4i ), whereas overexpressing SP1 increased FZD10 mRNA by 2.4-fold ( Fig. 4j ), suggesting that SP1-mediated transcription is responsible for FZD10 upregulation in breast cancer cells. Next, we evaluated whether SP1 binds to the potential SP1-binding site in FZD10 promoter using a ChIP assay with primers spanning SP1-binding site ( Supplementary Fig. 4d ). Anti-SP1 antibody efficiently retrieved the SP1-binding region but not the control distal region of FZD10 promoter in both MDA-MB-231 ( Fig. 4k ) and T47D cells ( Fig. 4l ). More importantly, enforcing BRMS1L expression in MDA-MB-231 cells notably reduced enrichment of the SP1-binding region ( Fig. 4m ), but not the control distal region of FZD10 promoter ( Supplementary Fig. 4e ), by anti-SP1 antibody, whereas silencing BRMS1L expression in T47D cells specifically increased enrichment of SP1-binding region ( Fig. 4n ), but not the distal region ( Supplementary Fig. 4f ). Therefore, SP1 is responsible for increased FZD10 transcription in breast cancer cells, whereas BRMS1L attenuates SP1-mediated FZD10 transcriptional activation probably by reducing histone acetylation at FZD10 promoter and thus suppressing SP1 recruitment to its binding site. BRMS1L inhibits Wnt pathway via suppressing WNT3-FZD10 As FZD10 is a cell-surface receptor for Wnt signalling, we investigated whether BRMS1L influences the activation of Wnt pathway in breast cancer cells via FZD10. Ectopic BRMS1L expression in MDA-MB-231 cells markedly reduced the mRNA level of AXIN2 and TCF-1 ( Supplementary Fig. 5a ), target genes of canonical Wnt pathway, and inhibited TCF/LEF luciferase activity ( Fig. 5a ), a hallmark of canonical Wnt activation. Conversely, RNA interference-mediated silencing of BRMS1L in T47D cells increased AXIN2 and TCF-1 expression ( Supplementary Fig. 5b ) and elevated TCF/LEF activity ( Fig. 5a ). However, modifying BRMS1L expression did not influence Jun N-terminal kinase (JNK) activation, hallmarks of non-canonical Wnt activation ( Supplementary Fig. 5c and d ). Furthermore, rescuing FZD10 expression attenuated downregulation of AXIN2 and TCF-1 ( Supplementary Fig. 5e ) as well as reduction in TCF/LEF luciferase activity ( Fig. 5b ) induced by BRMS1L overexpression in MDA-MB-231 cells. On the other hand, silencing FZD10 in T47D cells efficiently alleviated upregulation of AXIN2 and TCF-1 ( Supplementary Fig. 5f ) as well as elevation of TCF/LEF activity ( Fig. 5c ) induced by BRMS1L-siRNA. In addition, similar results were obtained by fractionation assay for nuclear translocation of β-catenin ( Supplementary Fig. 5g and Fig. 5d,e ), another marker for canonical Wnt pathway activation. 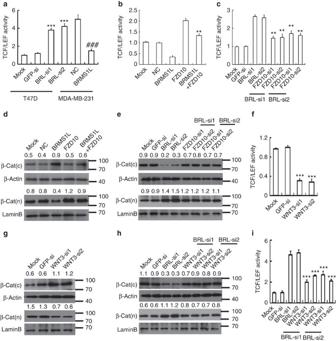Collectively, these data suggest that BRMS1L inhibits the activation of canonical Wnt/β-catenin pathway by suppressing FZD10 expression. Figure 5: BRMS1L suppresses WNT3/FZD10/β-catenin pathway. (a) Wnt/β-catenin activity measured by TCF/LEF luciferase reporter assays in T47D cells that were mock transfected (mock), or transfected with GFP-siRNA or two BRMS1L-siRNAs and in MDA-MB-231 cells that were transfected with pcDNA3 vector carrying BRMS1L (BRMS1L) or negative control (NC). Bars correspond to mean±s.d., ***P≪0.001 as compared with GFP-siRNA,###P≪0.001 as compared with NC. (b,c) Wnt/β-catenin activities measured by TCF/LEF luciferase assays in MDA-MB-231 (b) and T47D cells (c) treated as indicated. Bars correspond to mean±s.d. **P≪0.001 as compared with BRMS1L or BRMS1L-siRNA1. (d,e) Western blotting for nuclear (n) and cytoplasm (c) β-catenin in MDA-MB-231 (d) and T47D cells (e) treated as indicated. (f,g) Wnt/β-catenin activities measured by TCF/LEF luciferase assays (f) and β-catenin translocation (g) in MDA-MB-231cells treated as indicated. ***P≪0.001 as compared with GFP-siRNA. (h,i) Wnt/β-catenin activities measured by TCF/LEF β-catenin translocation (h) and luciferase assays (i) in T47D cells treated as indicated. ***P≪0.001 as compared with BRMS1L-siRNA1. β-cat, β-catenin; BRL, BRMS1L. Bars correspond to mean±s.d. These data are representative of three independent experiments. Student’st-test was used for the comparison of two independent groups ina,b,c,f,i. Figure 5: BRMS1L suppresses WNT3/FZD10/β-catenin pathway. ( a ) Wnt/β-catenin activity measured by TCF/LEF luciferase reporter assays in T47D cells that were mock transfected (mock), or transfected with GFP-siRNA or two BRMS1L-siRNAs and in MDA-MB-231 cells that were transfected with pcDNA3 vector carrying BRMS1L (BRMS1L) or negative control (NC). Bars correspond to mean±s.d., *** P ≪ 0.001 as compared with GFP-siRNA, ### P ≪ 0.001 as compared with NC. ( b , c ) Wnt/β-catenin activities measured by TCF/LEF luciferase assays in MDA-MB-231 ( b ) and T47D cells ( c ) treated as indicated. Bars correspond to mean±s.d. ** P ≪ 0.001 as compared with BRMS1L or BRMS1L-siRNA1. ( d , e ) Western blotting for nuclear (n) and cytoplasm (c) β-catenin in MDA-MB-231 ( d ) and T47D cells ( e ) treated as indicated. ( f , g ) Wnt/β-catenin activities measured by TCF/LEF luciferase assays ( f ) and β-catenin translocation ( g ) in MDA-MB-231cells treated as indicated. *** P ≪ 0.001 as compared with GFP-siRNA. ( h , i ) Wnt/β-catenin activities measured by TCF/LEF β-catenin translocation ( h ) and luciferase assays ( i ) in T47D cells treated as indicated. *** P ≪ 0.001 as compared with BRMS1L-siRNA1. β-cat, β-catenin; BRL, BRMS1L. Bars correspond to mean±s.d. These data are representative of three independent experiments. Student’s t -test was used for the comparison of two independent groups in a , b , c , f , i . Full size image We next determined which Wnt ligands are responsible for activation of canonical Wnt pathway via FZD10 in breast cancer cells with low BRMS1L expression. Out of 19 Wnt ligands that we screened, basal expression of WNT3, WNT4, WNT7B and WNT10B were high in MDA-MB-231 cells with low BRMS1L level ( Supplementary Fig. 6a ) and were upregulated in T47D cells after silencing BRMS1L ( Supplementary Fig. 6b ). However, only silencing of WNT3 ( Supplementary Fig. 7a ), but not WNT4, WNT7B and WNT10B ( Supplementary Fig. 7c,e and g ), significantly inhibited the expression of Wnt target genes, including AXIN2 and TCF-1, in MDA-MB-231 cells. Similar results were obtained in T47D cells with silenced BRMS1L ( Supplementary Fig. 7b,d,f,g and h ), suggesting that WNT3 could be the ligand that induces Wnt pathway activation in MDA-MB-231 cells with low BRMS1L expression and in T47D cells with BRMS1L knockdown. These findings were confirmed by examining TCF/LEF activity ( Fig. 5f ) and β-catenin nuclear translocation to determine canonical Wnt pathway activation in MDA-MB-231 cells ( Fig. 5g ) or in T47D cells transfected with BRMS1L-siRNA ( Fig. 5h,i ). Therefore, WNT3–FZD10 interaction contributes to canonical Wnt pathway activation in breast cancer cells with reduced BRMS1L. Increased miR-106b in mesenchymal-like cells silences BRMS1L To investigate whether reduced BRMS1L expression in mesenchymal-like breast cancer cells is due to transcriptional inhibition, a 2,015-bp DNA fragment between −1,959 to +56 relative to BRMS1L TSS was cloned into luciferase reporter pGL3-basic plasmid and transfected it into MCF-10A, T47D, BT474, MCF-7, MDA-MB-436 and MDA-MB-231 cells with different BRMS1L expression. However, luciferase activity was not significantly different among these cell lines ( Supplementary Fig. 8a ), indicating that transcription is unlikely to be the cause of different BRMS1L expression between epithelial- and mesenchymal-like breast cancer cells. To further evaluate posttranscriptional regulation of BRMS1L expression in breast cancer cells, we employed the miRNA Target Scan to screen for possible miRNA target sequences at the 3′ untranslated region (UTR) of BRMS1L. Herein, we identified seven miRNA target sequences ( Supplementary Table 5 ), and thus constructed a pMIR-REPORT reporter vector containing the 3′ UTR site of BRMS1L for validation. Among these seven miRNAs, miR-106b mimics was the most efficient to inhibit luciferase activity upon co-transfection with pMIR-REPORT containing BRMS1L-3′ UTR in 293T cells ( P ≪ 0.001, Fig. 6a ). In addition, miR-106b expression was much higher in primary breast cancers with LN metastasis (four cases) than those without metastasis (four cases; Fig. 6b ), which is opposite to the expression pattern of BRMS1L ( Fig. 1b ). In agreement with the luciferase reporter assay, miR-106b mimics significantly silenced BRMS1L mRNA and protein expression ( Supplementary Fig. 8b and c ) in T47D cells. Moreover, transfection of MDA-MB-231 cells with miR-106b antisense oligonucleotide significantly increased BRMS1L mRNA and protein expression ( Supplementary Fig. 8b and c ). 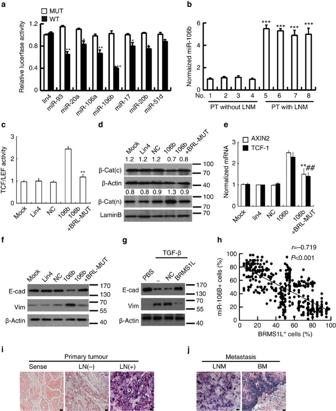These data suggested that miR-106b post-transcriptionally inhibits BRMS1L expression probably by degrading BRMS1L mRNA and inhibiting BRMS1L translation. Figure 6: miR-106b suppresses Wnt signalling pathway by targeting BRMS1L. (a) Luciferase reporter assays for 293T cells co-transfected with pMIR-REPORT reporter vector carrying the 3′ UTR of BRMS1L mRNA with wild-type (WT) or mutated (MUT) target site with microRNA mimics or lin4. *P≪0.05, **P≪0.01, ***P≪0.001 as compared with MUT. Bars correspond to mean±s.d.. These data are representative of three independent experiments. Student’st-test was used for the comparison of two independent groups. (b) qRT–PCR for miR-106b expression in primary breast tumour cells (PT) with or without lymph nodes metastasis (LNM;n=4 per group). Bars correspond to mean±s.d. Eight independent experiment were repeated (each patient sample was considered as one independent experiment. Five technological replications were repeated in each sample.). Student’st-test was used for the comparison of two independent groups. (c–e) Wnt/β-catenin activity measured by TCF/LEF luciferase reporter assay (c) and β-catenin translocation (d) and wnt target gene expression using qRT–PCR (e) in T47D cells that were mock transfected (mock), or transfected with lin4 mimics (lin4), an empty vector as negative control (NC), miR-106b mimics (106b), or co-transfected with miR-106b mimics and a vector carrying BRMS1L with a mutated miR-106b-target site at its 3′ UTR (BRMS1L-MUT). Bars correspond to mean±s.d., **P≪0.01 and##P≪0.01 as compared with 106b. Bars correspond to mean±s.d. The data are representative of three independent experiments. Student’st-test was used for the comparison of two independent groups. (f,g) Western blotting of E-cadherin and vimentin for T47D cells treated as inc(f) or treated with PBS or TGF-β (g). (h) Correlation between the percentages of BRMS1L+and miR-106b+breast cancer cells. BRL, BRMS1L. Linear regression was used to analyse the correlation. (i,j)In situhybridization (ISH) staining for miR-106b in primary breast cancers with or without regional lymph node (LN) metastasis (i), scale bar corresponds to 20 μm, as well as metastatic lymph nodes (LNM) and brain metastasis (BM;j), scale bar corresponds to 50 μm. Sense, using sense probe; other group, using antisense probe. E-cad, E-cadherin; Vim, vimentin; β-cat, β-catenin; BRL, BRMS1L. Figure 6: miR-106b suppresses Wnt signalling pathway by targeting BRMS1L. ( a ) Luciferase reporter assays for 293T cells co-transfected with pMIR-REPORT reporter vector carrying the 3′ UTR of BRMS1L mRNA with wild-type (WT) or mutated (MUT) target site with microRNA mimics or lin4. * P ≪ 0.05, ** P ≪ 0.01, *** P ≪ 0.001 as compared with MUT. Bars correspond to mean±s.d.. These data are representative of three independent experiments. Student’s t -test was used for the comparison of two independent groups. ( b ) qRT–PCR for miR-106b expression in primary breast tumour cells (PT) with or without lymph nodes metastasis (LNM; n =4 per group). Bars correspond to mean±s.d. Eight independent experiment were repeated (each patient sample was considered as one independent experiment. Five technological replications were repeated in each sample.). Student’s t -test was used for the comparison of two independent groups. ( c–e ) Wnt/β-catenin activity measured by TCF/LEF luciferase reporter assay ( c ) and β-catenin translocation ( d ) and wnt target gene expression using qRT–PCR ( e ) in T47D cells that were mock transfected (mock), or transfected with lin4 mimics (lin4), an empty vector as negative control (NC), miR-106b mimics (106b), or co-transfected with miR-106b mimics and a vector carrying BRMS1L with a mutated miR-106b-target site at its 3′ UTR (BRMS1L-MUT). Bars correspond to mean±s.d., ** P ≪ 0.01 and ## P ≪ 0.01 as compared with 106b. Bars correspond to mean±s.d. The data are representative of three independent experiments. Student’s t -test was used for the comparison of two independent groups. ( f , g ) Western blotting of E-cadherin and vimentin for T47D cells treated as in c ( f ) or treated with PBS or TGF-β ( g ). ( h ) Correlation between the percentages of BRMS1L + and miR-106b + breast cancer cells. BRL, BRMS1L. Linear regression was used to analyse the correlation. ( i , j ) In situ hybridization (ISH) staining for miR-106b in primary breast cancers with or without regional lymph node (LN) metastasis ( i ), scale bar corresponds to 20 μm, as well as metastatic lymph nodes (LNM) and brain metastasis (BM; j ), scale bar corresponds to 50 μm. Sense, using sense probe; other group, using antisense probe. E-cad, E-cadherin; Vim, vimentin; β-cat, β-catenin; BRL, BRMS1L. Full size image Next, we investigated whether miR-106b-mediated BRMS1L reduction is responsible for Wnt pathway activation and the ensuing EMT in breast cancer cells. Indeed, trasnfection of T47D cells with miR-106b mimics increased TCF/LEF activity, induced nuclear translocation of β-catenin and enhanced AXIN2 and TCF-1 expression ( Fig. 6c–e ), which could be reversed by ectopic expression of BRMS1L with a mutated miR-106b target site at its 3′ UTR. These data suggested that miR-106b activates Wnt/β-catenin signalling by silencing BRMS1L in breast cancer cells. Moreover, EMT induced by miR-106b mimics in T47D could be reversed by transfection of BRMS1L-expressing vector with a mutated miR-106b target site at its 3′ UTR ( Fig. 6f ). As our recent study has demonstrated that miR-106b is upregulated by transforming growth factor (TGF)-β in breast cancer cells [38] , which regulates EMT of breast epithelial cells, we further evaluated the influence of miR-106b-mediated BRMS1L reduction on TGF-β effects. Ectopic BRMS1L expression partially reversed TGF-β-induced EMT ( Fig. 6g ) of T47D cells, suggesting that excessive BRMS1L may antagonize the pro-tumour effects of TGF-β. To further understand the clinical relevance of miR-106b-induced BRMS1L reduction in breast cancer, we employed in situ hybridization to study miR-106b expression in breast cancer tissues. The percentage of miR-106b + cells was inversely correlated with that of BRMS1L + cells ( r =−0.719, P ≪ 0.001, Fig. 6h ). In addition, miR-106b expression was significantly higher in the tumour cells of primary breast cancers with regional lymph node metastasis than those without metastasis ( Fig. 6i ). Meanwhile, strong miR-106b signals were observed in cancer cells of metastatic lymph node and brain metastasis ( Fig. 6j ). Therefore, miR-106b-mediated BRMS1L reduction plays an important role in Wnt signal activation and EMT induction in breast cancer. BRMS1L inhibits metastasis of breast cancer in xenografts To determine the influence of BRMS1L on breast cancer metastasis, we established BT-474 cells that were enforced to stably express two short hairpin RNAs (shRNAs) targeting BRMS1L or green fluorescent protein (GFP) as negative control and MDA-MB231 cells stably overxpressing BRMS1L or negative control. Female nude mice ( n =8 per group) were inoculated in their mammary fat pads with BT-474 cells with GFP-shRNA or two BRMS1L-shRNAs (5 × 10 6 ), or MDA-MB-231 cells with control or BRMS1L expression vector (2 × 10 6 ). Although BRMS1L did not obviously change the primary tumour growth rate in these groups ( Supplementary Fig. 9a and b ), it increased the number of mice with liver metastases ( Supplementary Table 6 ), but no metastasis was found in the lung. Knockdown of BRMS1L in BT-474 cells significantly increased the number of metastatic nodules and human hypoxanthine-guanine-phosphoribosyltransferase (HPRT) mRNA in the livers, whereas overexpression of BRMS1L in MDA-MB-231 cells markedly reduced the number of liver metastatic nodules and HPRT mRNA ( P ≪ 0.001, t -test, Fig. 7a and b ). Figure 7: BRMS1L inhibits liver metastasis of breast tumour xenografts without influencing orthotopic tumour incidence and growth rate. ( a ) The number of metastatic liver nodules in mice xenografted with breast cancer cells as indicated. The bars correspond to the mean±s.d. *** P ≪ 0.001 compared with GFP-shRNA. ### P ≪ 0.001 as compared with NC ( n =8 per group). Student’s t -test was used for the comparison of two independent groups. ( b ) Expression of human HPRT mRNA relative to mouse 18S rRNA in the liver. Bars correspond to mean±s.d. Eight independent experiments were repeated (each mouse sample was considered as one independent experiment. Five technological replications were repeated in each sample.). Student’s t -test was used for the comparison of two independent groups. ( c ) Haematoxylin and eosin (H&E) staining for tumour xenografts and liver metastases of mice xenografted with breast cancer cells as indicated. Scale bars correspond to 50 μm. ( d ) Immunohistochemical staining for BRMS1L and FZD10 expression in tumour xenografts of mice xenografted with breast cancer cells as indicated. Scale bars correspond to 50 μm.BRL, BRMS1L. Full size image Haematoxylin and eosin staining also indicated that knockdown of BRMS1L led to massive metastasis in the liver compared with the control group ( Fig. 7c ). Conversely, overexpressing BRMS1L resulted in less liver metastasis ( Supplementary Table 6 , Fig. 7c and Supplementary Fig. 9c and d ). Therefore, BRMS1L inhibits metastasis of breast cancer in xenografts without influencing orthotopic tumour incidence and growth rate. To further determine whether BRMS1L regulates the expression of FZD10 in vivo , we examined protein levels in the xenografts using IHC. Knockdown of BRMS1L significantly increased FZD10 protein expression in the BT-474 xenografts, whereas ectopic BRMS1L efficiently decreased FZD10 protein expression in the MDA-MB-231 xenografts ( Fig. 7d ). Taken together, these results suggest that BRMS1L suppresses metastasis of breast cancer in xenografts without influencing orthotopic tumour incidence and growth rate and BRMS1L upregulation is associated with reduced FZD10 level in vivo . Histone deacetylation mediated by HDAC is a critical event in epigenetic silencing of target genes and thus plays an essential role in diverse pathological processes including cancer metastasis [39] , [40] . Recruitment of HDAC to the promoter regions of target genes is tightly regulated by proteins known as gene co-repressors. Here we demonstrated that BRMS1L, a newly identified component of the Sin3A co-repressor complex, suppresses invasion and metastasis of breast cancer cells by inhibiting EMT. The biological effect of BRMS1L is mediated by epigenetic silence of FZD10 gene by facilitating the recruitment HDAC1 to its promoter and enhancing histone H3K9 deacetylation. Furthermore, BRMS1L expression in breast cancer is associated with less metastasis and better clinical outcome. These findings highlight the contribution of BRMS1L in epigenetic silencing of oncogenes and its effect in tumour suppression. To our knowledge, BRMS1L is the second component in the Sin3A complex that has been shown to inhibit breast cancer metastasis following the characterization of BRMS1 (ref. 10 ). The tumour inhibitory effect of BRMS1L is potent, as it effectively suppresses the motility and invasiveness of breast cancer cells. However, similar to BRMS1, BRMS1L does not significantly influence proliferation of breast cancer cells, whereas it inhibits EMT of cancer cells, a key process in the cascade of metastasis. As BRMS1L is highly homologous to BRMS1 in the amino-acid sequence and preserves the Sds3-like domain for protein interaction, BRMS1L may compensate or augment the function of BRMS1, when the latter is genetically deleted or epigenetically silenced. On the other hand, although both BRMS1L and BRMS1 suppress gene expression by facilitating the recruitment of HDACs to the promoter regions and inducing chromosomal histone deacetylation, their target genes are different. BRMS1 has been shown to silence several receptors for metastasis-associated chemokines and growth factors, including urokinase-type plasminogene activator, EGFR and CXCR4, whereas BRMS1L inhibits the expression of FZD10, a receptor for Wnt/β-catenin signalling in cancer cells. Therefore, BRMS1L and BRMS1 may act synergistically to suppress breast cancer metastasis by inhibiting different cellular signalling pathways, respectively. Our findings that BRMS1L silences the expression of FZD10, a seven-transmembrane receptor for the Wnt/β-catenin pathway, suggest a link between BRMS1L and the Wnt pathway. Wnt signalling pathway has been shown to control self-renewal and differentiation of cancer cells [29] , and aberrant activation of Wnt signalling leads to EMT in breast epithelial cells [41] , [42] . As a receptor for the Wnt pathway, FZD10 is expressed at high level in colorectal cancers, gastric cancers, as well as in synovial sarcomas, and is associated with the activation of Wnt signalling in these cancers [33] , [34] , [43] . For instance, FZD10 activates the non-canonical Wnt/JNK pathway in synovial sarcoma cell [34] and enhances their anchorage-independent growth. On the other hand, FZD10 can activate the canonical Wnt/β-catenin/TCF signalling pathway in colorectal cancer cells [44] . Herein, we show that FZD10 overexpression in breast cancer cells due to reduced BRMS1L level leads to aberrant activation of canonical Wnt signalling and thus induces EMT in these cells. Moreover, our data are confirmed by Oncomine database demonstrating BRMS1L expression is negatively correlated with FZD10 and BRMS1L downregulation predicts poor prognosis for breast cancer patients. Moreover, BRMS1L is reduced and FZD10 is increased in triple negative breast cancers than the other subtypes, along with EMT phenotype with reduced E-cadherin and increased Vimentin, as well as elevated expression of Wnt target genes including β-catenin, TCF-1 and AXIN2 ( Supplementary Table 3 ). However, BRMS1L is not the only component in the Sin3A complex that regulate the activation of Wnt pathway. Others have showed that Sin3A complex may enhances degradation of β-catenin by regulating PP1 transcription and thus inhibits overactivation of Wnt/β-catenin signalling [45] . Therefore, components of the Sin3A co-repressor complex may work synergistically to modulate the activity of Wnt signalling at different levels. Furthermore, previous study had shown that a humanized antibody against FZD10 might serve as a promising therapy for patients with tumours overexpressing FZD10 (ref. 46 ). Our present study may suggest that restoring the expression of BRMS1L in breast cancer cells may be of therapeutic potential by transcriptionally downregulating FZD10 and inhibiting overactivation of the Wnt/β-catenin signalling. It has been shown that BRMS1 locates at the chromosome region with high incidence of deletion, suggesting that loss of BRMS1 in cancer cells is mainly attributed to genetic deletion [47] . In contrast, our present study showed that reduced BRMS1L expression in advanced breast cancers is due to miR-106b upregulation. Inhibiting miR-106b by antisense oligonucleotides successfully restored BRMS1L expression and inhibits EMT in breast cancer cells. Our recent study and others have shown that miR-106b overexpression in breast cancers correlates with tumour metastasis and poor patient outcome [38] , [48] . Moreover, miR-106b is a potent oncomiR that has been shown to target and silence a list of tumour-suppressing genes, including Rb [49] , smad7 (ref. 48 ), PTEN [50] and thus promote the proliferation and invasion of cancer cells. Our present study has extended this list by showing that metastasis-suppressing BRMS1L is also a target of miR-106b, and via BRMS1L the miRNA regulates the activation of Wnt pathway. Although it was reported that miR-106b may induce EMT in breast cancer cells by targeting Smad7, an inhibitor of the Smad pathway, and thus activate TGF-β signalling [51] , our present findings that miR-106b-mediated downregulation of BRMS1L also induces EMT in breast epithelial cells has linked the miRNA to the activation of Wnt signalling. Hence, miR-106b may regulate EMT via both the TGF-β pathway and the canonical Wnt/β-catenin pathway. In summary, our present study has highlighted the importance of a new signalling pathway formed by miR-106b, BRMS1L and FZD10, which promotes breast cancer metastasis by inducing EMT of breast cancer cells ( Fig. 8 ). As a central link of this axis, BRMS1L downregulation may not only serve as a prognostic factor to predict clinical outcome for breast cancer patients, but also a therapeutic target as ectopic BRMS1L expression efficiently inhibits breast cancer metastasis by suppressing the activity of Wnt signalling. 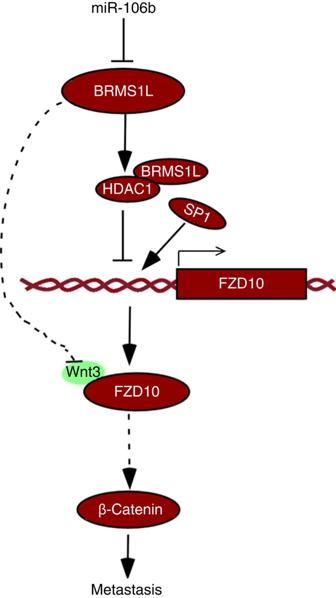Figure 8: Schematic summary of the miR106b-BRMS1L-FZD10 signalling pathway.  Figure 8: Schematic summary of the miR106b-BRMS1L-FZD10 signalling pathway. Full size image Patients and tissue samples Primary invasive ductal carcinomas of breast were obtained from 428 female patients with a medium age of 45.5 years at the Breast Tumor Center, Sun Yat-Sen Memorial Hospital, Sun Yat-Sen University, from January 2007 to October 2012. Pathological diagnosis, as well as estrogen receptor/PR and Her2 status, was verified by two different pathologists. No distal metastasis was identified in the patients upon diagnosis. Seventy-eight cases developed distant metastasis during follow-up. In addition, fresh samples of normal breast tissue, invasive ductal carcinoma and metastatic lymph nodes were collected from patients who undergone mastectomy or lumpectomy for benign or malignant breast diseases. Metastatic lesions were obtained via surgery or biopsy. The primary breast cancer tissues matched with the metastasis. All samples were snap-frozen for mRNA assessment and were collected with informed written consent from patients. All related procedures were performed with the approval of the Internal Review and the Ethics Boards of the Sun Yat-Sen Memorial Hospital. Cell cultures and treatment MCF-7, T47D, ZR75-1, BT-474, MDA-MB-453, BT-549, MDA-MB-231 and MDA-MB-436 breast cancer cell lines as well as MCF-10A breast epithelial line were obtained from American Type Culture Collection and cultured according to the recommended protocols. For siRNA and stable plasmid DNA transfection, cells were transfected with specific siRNA duplexes targeting BRMS1L or FZD10 or pcDNA3 vector expressing BRMS1L or FZD10 construct using Lipofectamine 2000 (Invitrogen) according to the manufacturer’s instruction. To inhibit HDAC activities, cells were treated with 200 ng ml −1 trichostatin A (Sigma) for 24 h. Immunohistochemistry IHC was performed on paraffin sections of breast tissues according to the standard LSAB protocol (Dako), using primary antibodies against BRMS1L (1:200, NBP2-14362, Novus), FZD10 (1:200, NBP1-00826, Novus). Isotype-matched IgG was used as negative controls. BRMS1L expression level was scored semiquantitatively using the IRS=SI (staining intensity) × PP (percentage of positive cells) as described [52] , [53] . Briefly, SI was determined as 0, negative; 1, weak; 2, moderate and 3, strong. PP was defined as 0, ≪ 1%; 1, 1–10%; 2, 11–50%; 3, 51–80% and 4, >80% positive cells. Ten visual fields from different areas of each tumour were used for the IRS evaluation. IRS≤4 was defined as low BRMS1L expression and IRS>4 were defined as high BRMS1L expression. In situ hybridization and data analysis Formalin-fixed, paraffin-embedded sections of breast cancer tissues were obtained from the Breast Tumor Center at Sun Yat-Sen Memorial Hospital. Following wax removal and rehydration, the samples were digested with Proteinase K, hybridized with the 5′ digoxin-labelled, Locked Nucleic Acid-modified miR-106b probe (Exiqon) at 49.5 °C overnight and then incubated overnight at 4 °C with an anti-digoxin monoclonal antibody (Roche). After treatment with an NBT/BCIP staining solution in the dark and counterstaining with nuclear fast red, the sections were mounted and observed. The staining was scored by combining the proportion of positively stained tumour cells and the intensity of staining. A Staining Index (SI) score of 4 was used as a cutoff value based on the distribution of the frequency of the SI scores for miR-106b expression, and the expression levels of miR-106b were defined as high (SI>4) or low (SI≤4). Immunofluorescence For immunofluorescent staining, the cells were incubated with primary antibodies against E-cadherin (1:100, 3195S, CST), vimentin (1:200, AF2105, R&D) or β-catenin (1:1,000, ab16051, Abcam) followed by incubation with Alexa488-conjugated goat antibody against rabbit (1:100, A11008, Life) or Alexa594-conjugated rabbit antibody against goat (1:100, A11080, Life). For confocal microscopy, cells on coverslips were counterstained with 4,6-diamidino-2-phenylindole and imaged using a confocal laser-scanning microscope (Carl Zeiss) with a core data acquisition system (Applied Precision). Boyden chamber assay Invasion and migration of breast cancer cells were examined using 24-well Boyden chambers (Corning) with 8 μM inserts with or without precoated Matrigel Basement Membrane Matrix (BD Biosciences), respectively. Breast cancer cells (10 5 cells per well) were placed on the inserts in the upper chambers and cultured at 37 °C in 5% CO 2 . After 8 h (migration assay) or 18 h (invasion assay), cells on the upper surface of the membrane filter were removed. The migrated and invaded cells that crossed the inserts to the lower surface were fixed with 4% formaldehyde, stained with crystal violet (0.005%, sigma), and counted as cells per field of view under phase-contrast microscopy. Wound-healing assay Breast cancer cells were cultured under permissive condition to about 90% confluence. A linear wound was created in the confluent monolayer using a pipette tip. Cancer cells were allowed to close the wound for 12 h, and observed under phase-contrast microscopy. The scratch width per viewfield at 0 and 12 h following wound closure was determined using the Carnoy software (Biovolution), and the percentage of wound closure indicated by scratch width reduction within 12 h was assessed. mRNA microarray analysis mRNA array analysis was performed in MDA-MB-231 cells transfected with either pcDNA3 vector carrying BRMS1L or an empty vector as negative control. Two pairs of independent samples were used for mRNA array analysis. After transfection for 24 h, total RNA was harvested using Trizol (Invitrogen) according to the manufacturer’s instructions. Total RNA from each sample was quantified by NanoDrop ND-1000 (ThermoFisher) and RNA integrity was accessed by standard denaturing agarose gel electrophoresis. Reverse transcription for first strand cDNAs were synthesized using Invitrogen Superscript ds-cDNA synthesis kit (Invitrogen). The ds-cDNA samples were labelled according to the manufacturer’s instructions (Kangchen). Array scanning was performed with an Axon GenePix 4000B microarray scanner (Molecular Devices Corporation). Scanned images (TIFF format) were then imported into NimbleScan software (version 2.5) for grid alignment and expression data analysis. Expression data were normalized through quantile normalization and the Robust Multichip Average (RMA) algorithm included in the NimbleScan software. The Probe level (*_norm_RMA.pair) files and Gene level (*_RMA.calls) files were generated after normalization. The two gene level files were imported into Agilent GeneSpring GX software (version 11.5.1) for further analysis. Genes with values above the cutoff of 100.0 in all samples (‘All Targets Value’) were chosen for data analysis. Differentially expressed genes were identified through Fold Change filtering. Pathway analysis and GO analysis were applied to determine the roles of these differentially expressed genes played in these biological pathways or GO terms. Finally, Hierarchical Clustering was performed to show distinguishable gene expression profiling among samples. Western blotting Protein extracts were resolved in 8–15% SDS–polyacrylamide gel electrophoresis, transferred to polyvinylidene difluoride membranes and probed with antibodies against E-cadherin (1:1,000, 3195S, CST), vimentin (1:1,000, AF2105, R&D), BRMS1L (1:1,000, NBP2-14362, Novus), FZD10 (1:500, NBP1-00826, Novus), JNK (1:1,000, 9258, CST), p-JNK (1:1,000, Thr183/Tyr185, 4668S, CST), β-catenin (1:4,000, ab16051, Abcam) and β-actin (1:25,000, A3854, Sigma). Peroxidase-conjugated secondary antibodies against mouse (1:40,000, A0168, Sigma), rabbit (1:40,000, A0545, Sigma), goat (1:40,000, A5420, Sigma) were used, and the antigen–antibody reaction was visualized by the enhanced chemiluminescence assay (WBKLS0500, Millipore). To obtain the β-catenin protein extracts, the nuclear and cytoplasm β-catenin were isolated, respectively, using subcellular protein fractionation kit (78840, Thermo). The original blot images of western blotting analysis are shown in Supplementary Fig. 10 . ChIP assay MDA-MB-231 cells were transfected with Myc-taged BRMS1L or negative control for 24 h. T47D cells were transfected with BRMS1L-siRNAs or GFP-siRNA for 72 h. Cells were crosslinked in 1% formaldehyde solution for 10 min at room temperature, followed by the addition of 125 mM glycine for 5 min. ChIP assay was performed with ChIP assay kit (26156, Thermo) according to the manufacturer’s instructions. The nucleoprotein complexes were digested to yield DNA fragments ranging from 200 to 500 bp using the Micrococcal Nuclease in the kit. Two micrograms of normal IgG were used as the negative control, and anti-HDAC1 (17–608, Millipore), anti-acetyl histone H3K9 (17–658, Millipore), anti-SP1 (9389S, Cell signaling Technology, USA) and anti-Myc (SC-40AC, Santa Cruz) antibodies were used for each immunoprecipitation. The immunoprecipitates were eluted and reverse crosslinked, after which the DNA fragments were purified. Immunoprecipitated and input DNAs were subjected to qRT–PCR analysis. The primers used for amplifying the proximal promoter of FZD10 were forward: 5′- ATGGCCCAGGCTATAAAACG-3′ and reverse: 5′- GCCGAGGTTACGGGAAGTT-3′ . The primers used for amplifying FZD10 promoter region spanning SP1-binding site were forward: 5′- AAAGTTGGAGGCCAGGCAGA-3′ and reverse: 5′- CCGCTGCTTTGCATGAGAA-3′ . The primers used for amplifying the distal promoter of FZD10 were forward: 5′- TGTCATATTGCCCTAGTCCGA-3′ and reverse: 5′- CTGCTGCTCTGCTAACTCCTTC-3′ . The amount of immunoprecipitated DNA was normalized to the input DNA. Tumour xenografts Female nude mice were bred and maintained under defined conditions at the Animal Experiment Center of Sun Yat-Sen University, and all procedures were approved by the Animal Care and Use Committee of Sun Yat-Sen University and conformed to the legal mandates and national guidelines for the care and maintenance of laboratory animals. BT-474 cells (5 × 10 6 ) that were infected with lentivirus carrying GFP-shRNA or two BRMS1L-shRNAs, as well as MDA-MB-231 cells (2 × 10 6 ) that were infected with retrovirus vector pBABE-puro overexpressing BRMS1L or negative control were inoculated into the mammary fat pads of mice ( n =8 per group). Tumour growth was evaluated by monitoring tumour volume (TV=length × width 2 × 0.5) every 3 days for 8 weeks. When the xenografts became palpable (around 1.5 cm in diameter) the mice were killed, and their tumour xenografts, lungs and livers were harvested for further evaluation. Paraffin sections (4 μm) of harvested tissues were stained with haematoxylin and eosin for histological assessment, and total RNA was extracted for qRT–PCR analysis of human HPRT mRNA expression. Statistics All statistical analyses were done using SPSS for Windows version 16.0. Student’s t -test and one-way analysis of variance were used to correlate BRMS1L level with cancer metastasis, whereas χ 2 test was applied to analyse the association between BRMS1L expression and clinicopathological status. Kaplan–Meier survival curves were plotted, and log rank test was done. The significance of different variables for survival was analysed by the Cox proportional hazards model in a multivariate analysis. All experiments in vitro were performed independently for at least three times and in triplicate for each time. All results are expressed as mean±s.d., and mean values of three experiments are shown. Student’s t -test was used for the comparison of two independent groups. A P value ≪ 0.05 was considered statistically significant in all cases. How to cite this article: Gong, C. et al . BRMS1L suppresses breast cancer metastasis by inducing epigenetic silence of FZD10. Nat. Commun. 5:5406 doi: 10.1038/ncomms6406 (2014). Accession codes: Microarray data were deposited to GEO database with the accession code GSE61354 .